Experimental quantum key distribution with finite-key security analysis for noisy channels In quantum key distribution implementations, each session is typically chosen long enough so that the secret key rate approaches its asymptotic limit. However, this choice may be constrained by the physical scenario, as in the perspective use with satellites, where the passage of one terminal over the other is restricted to a few minutes. Here we demonstrate experimentally the extraction of secure keys leveraging an optimal design of the prepare-and-measure scheme, according to recent finite-key theoretical tight bounds. The experiment is performed in different channel conditions, and assuming two distinct attack models: individual attacks or general quantum attacks. The request on the number of exchanged qubits is then obtained as a function of the key size and of the ambient quantum bit error rate. The results indicate that viable conditions for effective symmetric, and even one-time-pad, cryptography are achievable. Quantum key distribution (QKD) is a technique for sharing a random secret key by means of a quantum link between two distant partners, traditionally called Alice and Bob. For this purpose, an optical link is established with Alice acting as the sender and Bob as the receiver in a prepare-and-measure scenario, or with both receiving a signal from an intermediate source [1] . The secret key that is obtained may be used in any symmetric cryptographic algorithm including the one-time-pad encryption introduced by Vernam [2] or computationally secure ciphers such as advanced encryption standard (AES). QKD may be considered the first successful example of a quantum information protocol that reached the everyday applications. Indeed, commercial devices communicating via optical cables are already operated worldwide. The perspective use in free space is also considered very attractive. This use includes terrestrial links, in the case that it is not possible to use optical cables, or in the case that either terminal is moving, including the very relevant case of key exchange with orbiting terminals, that is, satellite QKD. This extension of the QKD application has been fostered for years, being included in the major Quantum Information Roadmaps [3] , [4] , [5] , and has been the subject of several feasibility studies [6] , [7] , [8] , [9] , [10] , [11] , [12] . However, the intrinsic difficulties in its realization allowed only the experimental demonstration of the single-photon exchange with an orbiting terminal [13] . Moreover, in free-space links the gathering of light from the background is much more pronounced than for optical fibres. At the same time, in the case of long-distance terrestrial links or space to ground links, signal attenuation is typically greater by at least three orders of magnitude. As a consequence, strong noise overimposed to an attenuated signal results in a poor signal-to-noise ratio and in an increased quantum bit error rate (QBER) in the sifted key. The experimental investigation of such limit is therefore of crucial interest, to open the way to direct experiments in the free-space QKD, and the recent result on finite-key bounds by Tomamichel et al. [14] provides the necessary theoretical framework. As the final goal of this work, we aim to prove experimentally the bound for the number of exchanged raw key bits that is necessary to extract a secret key of desired length. This is the recipe needed to design the terminal dimension and performance in practical applications. Any QKD protocol consists of a physical quantum communication layer and a post-processing layer, in which, by using a classical communication channel, the secret key is extracted from the raw data shared by the two terminals: first, the raw data are sifted to distil maximally correlated data between Alice and Bob, then an information reconciliation protocol is performed to correct the errors between the two users and finally a privacy amplification algorithm is used to ensure the secrecy of the final key. A crucial parameter is the so-called secure key rate, that is, the ratio of the number of secret bits that can be extracted to the number of correlated, or raw, bits obtained in the quantum layer of the protocol. According to the standard QKD unconditional security proofs, the secret key rate is upper-bounded by the asymptotic limit that is achievable in the limit of infinitely long keys (see for example Scarani et al. [1] ), with the use of shorter blocks leading to lower key rates. However, in QKD implementations, the length of processed blocks is chosen as a trade-off between link duration constraints and memory resources on one side and efficiency (in terms of secret key rate) on the other. This trade-off usually results in long blocks, of at least a million sifted bits. However, in some scenarios such a choice may rather be constrained by the physical channel, as in the perspective use with satellites, where the passage of the orbiting terminal over the ground station is restricted to a few minutes in the case of low-earth-orbit satellite [13] , [9] or to a fraction of 1 h for the medium-earth-orbit ones [10] . Hence, for practical use of QKD in cryptography, it is of crucial importance to develop and test methods that give the achievable secure key rates in the bounded-key-length scenario, because the number of exchanged bits between the two parties is always finite. In the last years, great efforts from the quantum communication community were directed to this subject, because of its relevance for a number of application scenarios [15] , [16] , [17] , [18] , [19] , [20] , [21] . We would like to underline that all previous published experimental works on finite-size key security were based on a far more inefficient bound as compared with the one obtained in Tomamichel et al. [14] In this work, we study the security and the generation rate of a protocol for key exchange in the finite-key regime and in presence of noise, whose value is experimentally varied up to the top limit. The security is assessed with reference to a recently introduced theoretical result [14] , for which ‘almost tight bounds on the minimum value’ of exchanged qubits ‘required to achieve a given level of security’ were obtained [14] , as well as for a realistic bound described below. In particular, by leveraging the optimal design of the prepare-and-measure scheme complying with the above-mentioned tight theoretical bounds, we evaluate how the secret key rate scales in different channel conditions, depending on the protocol parameters. We consider two possible attack models, referring to two different levels of secrecy: ‘pragmatic secrecy’, which ensures resiliency against individual attacks, and ‘general secrecy’, which ensures resiliency against the most general quantum attacks. Protocol for QKD We will adopt here the protocol described in Tomamichel et al. [14] , a derivation of the well-known BB84 protocol [22] . According to this protocol, one of the two bases is used to encode the raw key bits, whereas the other basis is used to test the channel for the presence of the eavesdropper [23] . Moreover, the two bases are selected by Alice and Bob in the preparation of the qubits and in their measure, respectively, with non equal probabilities, unlike the standard BB84. Let us describe in more detail the quantum communication part of the QKD protocol used in the present experiment, characterized by the sifted key length n and the number of bits used for parameter estimation k ; both parameters can be chosen according to the required secret key length and channel conditions as described below. Alice prepares and sends to Bob quantum states encoded by means of photon polarization. She can choose between two bases, and with . For each basis, the first state represents the bit 0 and the second state represents the bit 1. Alice sends to Bob the raw key (namely a sequence of uniformly random bits) by randomly and asymmetrically encoding the bits with one of the two bases: with probability , she encodes the bits in the basis, and with probability p =1− p , she encodes the bits in the basis. Bob measures the photons by randomly choosing a basis, or , with the same probabilities p and p . Alice and Bob broadcast their basis choices over the classical channel, and Bob also communicates when he received the photons; bits corresponding to non-received photons are discarded. Otherwise, when Alice and Bob have both chosen the same basis (it happens with probability for the basis and with probability for the basis), they store the respective bits, whereas when they have chosen different bases, their bits are discarded. The protocol repeats the quantum communication as long as either the number of bits is lower than n or the number of bits is lower than k . To obtain the final sifted keys, Alice and Bob keep the same n bits, randomly chosen, from the bits to form the sifted key strings X ={ x i } and X′ ={ x ′ i }. Similarly, they choose k random bits from the bits to obtain the parameter estimation strings Z ={ z i } and Z′ ={ z ′ i }. Differently, from Tomamichel et al. [14] , we defined the sifted key as X and not as the union set of X and Z . The bits will be used to build the final secret key, and the expected number of errors between X and X′ is the crucial parameter in the design of the information reconciliation protocol. The bits will be used to test the presence of the eavesdropper, and the number of errors between Z and Z′ is used for dimensioning the privacy amplification procedure. Note that the probabilities p and p are chosen to satisfy to minimize the number of exchanged photons before the quantum communication is stopped. After the quantum transmission and the sifting of the raw data, four subsequent tasks take place: parameter estimation, information reconciliation, error verification and privacy amplification. The first task, parameter estimation, is required to measure the QBER on the basis, Q . Furthermore, we assume that the quantum channel is stable, that is, the QBER on the basis, Q , is constant in time (note that, in general, Q ≠ Q ). If Q increases (for instance because an attacker is tampering with the channel), then the information reconciliation will fail. The failure will be detected during the error verification phase, and the protocol will abort. On the other hand, the empirical QBER in the basis is dynamically computed at each protocol run as , to check for the presence of an eavesdropper. The protocol aborts if , where is a given channel error tolerance on the basis that has been determined a priori based on the expected behaviour of the quantum channel and the required level of security. Information reconciliation allows Bob to compute an estimate of X by revealing L EC bits ( L EC represents the classical information leakage). We define P fail as the upper bound to the probability of a reconciliation failure and ε cor as the upper bound to the probability that differs from X . We fixed a threshold such that the empirical QBER in the sifted key is higher than with probability < P fail /2. For details on the chosen information reconciliation, error verification and privacy amplification mechanisms, see the Methods section. General and pragmatic secrecy As introduced above, in this work we consider two possible attacker models, which in turn entail two different notions of secrecy, which we call ‘general’ and ‘pragmatic’, respectively. General secrecy, as defined in Tomamichel et al. [14] , requires that the final shared keys are secret with respect to the most general quantum attacks, and it is based on the secrecy criterion provided in König et al. [24] We say that the distilled key S is ε sec −GS (general secret) if for any attack strategy being || ρ || 1 =Tr , p abort the probability that the protocol aborts, ρ SE the quantum state that describes the correlation between classical key S of Alice and the eavesdropper, ω S the fully mixed state on S and σ E a generic quantum state on the eavesdropper’s Hilbert space. Then, if the bases and are chosen as described above and assuming that Alice uses an ideal single-photon source, Tomamichel et al. [14] show that an ε sec −GS key can be extracted out of the reconciled key, with length where , h 2 ( x )=− x log 2 x −(1− x )log 2 (1− x ) is the binary Shannon entropy function, ( x )= h 2 ( x ) for 0≤ x ≤0.5 and ( x )=1 for x >0.5. On the other hand, pragmatic secrecy [25] ensures that the final key is secret with respect to intercept-and-resend (IS) attacks [26] , that is, a specific class of selective individual attacks, which, however, represents the most realistic and feasible attack strategy based on the experimental technology nowadays available: collective or more general attack models (see Scarani et al. [1] ), in fact, require ancillary qubits and quantum memories to be deployed. Although in a long-term perspective (>50 years) general security is the goal, in the near future (5–10 years), we know that an ideal IS attack is the best option that an eavesdropper can choose because the quantum memory needed for a general or coherent attack is not yet available. In the Experimental results subsection, we will show that there are situations in which no key can be extracted if general security is required, whereas a pragmatically secure secret key can be obtained. In these cases, requiring general security, a protection far above actual possibilities of an eavesdropper, prevents key generation. Also, we would like to stress that pragmatic secrecy, unlike computational secrecy, offers forward security: if a key is produced today with pragmatic secrecy (without quantum memory available for Eve), the key or a message encrypted with it will be secure for any future use. As a criterion for pragmatic secrecy, we use a bound on the classical equivocation at the eavesdropper, namely we say that the distilled key S is δ sec −PS (pragmatic secret), for any IS attack strategy and in the case that the protocol is not aborting, being U S the uniform key with the same length as S , V the classical random variable that summarizes all the information available to the eavesdropper and H ( S | V ) the equivocation (conditional entropy) of S given V . Note that equation (3) implies the uniformity and the security conditions: where the accessible information I acc is the maximum mutual information I ( S ; V )= H ( S )− H ( S | V ) that can be extracted from the quantum system E (ref. 24 ). Moreover, choosing in equation (3) implies condition (1) for non-coherent attacks (see Methods section). It should be noted that, as for incoherent individual attacks, equation (3) guarantees composable security, as the eavesdropper, without a quantum memory, cannot exploit the ‘locking property’ of the accessible information (see König et al. [24] ). The pragmatic security of the distilled key can be assessed through the following result, the proof of which is provided in the Methods section. Theorem 1: The distilled key S is δ sec −PS if where with n EC = n − L EC −(log 2 ( P fail / ε cor )) and I x ( a , b ) denoting the regularized incomplete beta function (Abramowitz and Stegun [27] , section 6.6), Based on equation (5), we can therefore choose the optimal secret key length as Please note that, to allow a comparison with the tight bound (2), we have derived the secure key length in the hypothesis that Alice uses a single-photon source. Finally, given the probability ε rob that the protocol aborts even if the eavesdropper is inactive [14] , we can compute the final secret key rate for both general and pragmatic secrecy as: where M ( n , k )= n + k +2 is the expected number of qubits that have to be sent until n sifted key bits and k parameter estimation bits are collected. Experimental results We conducted experiments with different noisy channels yielding different values for the average QBERs Q and Q , each of them realized with different encoding probabilities ( p , p ). We varied the noise value in the channel by coupling to the receiver an external unpolarized source of suitable intensity, which increased the background signal. It is worth noting that by this operation we are modelling the following depolarizing channel: where σ j are the Pauli matrices, being σ 0 the identity and P the parameter representing the probability that any detected photon is coming from the background. In Fig. 1 , we show the joint empirical distribution of the transmitted and received bits on the and bases obtained in one run with the best environmental conditions (that is, with additional background), for the case p =49% and p =51%. As expected, in this case the QBER is very low: the main source of errors are imperfections in the waveplates used in the measurement, yielding Q =0.33% and Q =1.48% on average. 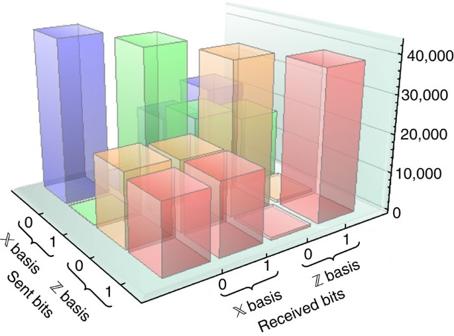Figure 1: Experimental bits. Joint empirical distribution of sent and received bits, as obtained in one experiment with the best channel conditions (corresponding toQ=0.33% andQ=1.48%). The probabilities of sending and measuring in theandbasis werep=0.51 andp=0.49, respectively. Figure 1: Experimental bits. Joint empirical distribution of sent and received bits, as obtained in one experiment with the best channel conditions (corresponding to Q =0.33% and Q =1.48%). The probabilities of sending and measuring in the and basis were p =0.51 and p =0.49, respectively. Full size image In Fig. 2 , we show the measured experimental key rates for each data set and for both general and pragmatic secrecy. First of all, let us recall that, to consistently compare the secrecy rates obtained with general and pragmatic secrecy, the security parameters ε sec and δ sec have to be chosen so that . As a performance reference, we plot the asymptotic theoretical bound r =1− h 2 ( Q )− h 2 ( Q ), holding in the limit of infinite length keys (labelled as ‘asymptotic’ in Fig. 2 ) and the optimal theoretical bound for ε sec −GS keys (labelled as ‘numerically optimized p ’ in Fig. 2 ). The experimental key rates are obtained by the following procedure: for each data set the n -bit sifted key X and the k -bit parameter estimation string Z ( X′ and Z′ ) at Alice’s (Bob’s) side are obtained by the experiment. The error correction is performed on X and X′ by using the Winnow scheme; in particular, the Winnow parameters were chosen so that a maximum of six subsequent iterations are allowed with block sizes up to 256 bits. We then performed privacy amplification by compressing the error-free keys by multiplication with a random binary Toeplitz matrix. The amount of compression depends on , the secret key length, given by equations (2) and (8) for general and pragmatic security, respectively. On the other hand, the optimal bound for ε sec −GS keys is numerically derived by maximizing the secret key rate r (equation (9), with given by equation (2)) over p , and for each n . 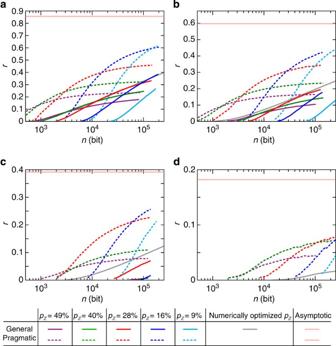Figure 2: Experimental key rates. Experimental secret key ratesrversus sifted key lengthnfor different probabilities of encoding and measuring on the two basesp,p=1−pand for different channel conditions (values of the average QBERsQ,Q): (a)Q=0.3%,Q=1.5%; (b)Q=2.4%,Q=3.9%; (c)Q=4.9%,Q=6.0%; and (d)Q=8.3%,Q=8.1%. For each case, we report the key rates obtained forεsec−GS (solid lines) andδsec−PS (dashed lines) keys withεsec=10−10,,Pfail=10−3and a correctness parameterεcor=10−10. The s.d. of experimental rates are on the order of 10−3for bothεsec−GS andδsec−PS keys. Error bars are not reported in the plot for the sake of clarity. For comparison, we also report the asymptotic key rate in the infinite length limit, and theεsec−GS is bound that is achievable by optimizing the probabilitypand the thresholdsfor each value ofn. Figure 2: Experimental key rates. Experimental secret key rates r versus sifted key length n for different probabilities of encoding and measuring on the two bases p , p =1− p and for different channel conditions (values of the average QBERs Q , Q ): ( a ) Q =0.3%, Q =1.5%; ( b ) Q =2.4%, Q =3.9%; ( c ) Q =4.9%, Q =6.0%; and ( d ) Q =8.3%, Q =8.1%. For each case, we report the key rates obtained for ε sec −GS (solid lines) and δ sec −PS (dashed lines) keys with ε sec =10 −10 , , P fail =10 −3 and a correctness parameter ε cor =10 −10 . The s.d. of experimental rates are on the order of 10 −3 for both ε sec −GS and δ sec −PS keys. Error bars are not reported in the plot for the sake of clarity. For comparison, we also report the asymptotic key rate in the infinite length limit, and the ε sec −GS is bound that is achievable by optimizing the probability p and the thresholds for each value of n . Full size image In the numerical procedure used to find the optimal bound for ε sec −GS keys, because an analytical expression is not available for L EC or ε rob , L EC is approximated as L EC =1.1· n · h 2 ( Q ) and, similarly, ε rob is replaced by the following upper bound (see equation A5 of Tomamichel et al. [28] for details): Experimental values obtained for ε rob show that such bound is rather loose. On the other hand, as Q increases, the approximate expression for L EC is lower than the average value for the Winnow scheme. As a consequence, the experimental secret key rates may slightly exceed the optimal bound in some low QBER cases, as we can see in Fig. 2a . As a further comment, we note that, for an asymmetric channel with Q < Q , using the basis for key encoding and for eavesdropper detection provides a higher optimal secret key rate (equation (9)). However, when the two error rates Q and Q have similar values, a minor gain in r is obtained. For instance, when n =10 6 , ε cor = ε sec =10 −10 , with Q =4% and Q =2%, we can achieve r =0.31; by exchanging the role of and , r =0.33 can be achieved. In situations such as satellite quantum communications, the amount of sifted bits is expected to fluctuate as it depends on the variable channel conditions during the passage. From the experimental point of view, it is easier to fix the values of p and p and accumulate data as long as possible. The value of p will constrain the ratio between k and n according to the relation . In the performed experiments, we thus fixed the value of p and p =1− p . For each value of the background noise, we run different acquisitions with p belonging to the discrete set {9%, 16%, 28%, 40%, 49%}. Experimental results for the ε sec −GS key rates are plotted with thin solid lines, whereas δ sec −PS key rates are plotted with thin dashed lines; different colours correspond to different ( p , p ). We used P fail =10 −3 , ε cor =10 −10 and ε sec =10 −10 . As expected, pragmatic secrecy always allows the achievement of higher secret key rates with respect to general secrecy, which pays the price for the higher level of secrecy it provides. The gain becomes more evident when the channel becomes noisier and the QBER increases. We also observe that with Q =4.9% ε sec −GS key securities are obtained for p =16%, p =28%, p =40% and p =49% and not for p =9%, whereas, when Q =8.3%, only keys that are secure against pragmatic secrecy can be extracted with the parameters we used. We point out that the bounds derived for the general and pragmatic secrecy do take into account statistical fluctuations: if the measured is greater than , protocol aborts, whereas for the protocol gives a secure key with security parameter ε sec . As an example, given Q =4.9%, Q =6.0%, n =100,000 and p =9%, the parameter μ that takes into account these fluctuations for general secrecy (see equation (2)) is approximately equal to 0.15, a value which, for an experimentally realistic number of bits disclosed during the information reconciliation procedure, and even without the contribution of , yields the impossibility of producing a secret key. Moreover, we notice that higher values of p (~50%) better suit lower values of n for both general and pragmatic secrecy in all considered cases: for instance, when Q =0.3% in the general secrecy case, p =49% is optimal for n <3 × 10 3 ; on the other hand, as n increases, it is possible to decrease p , and, when n ≃ 10 5 , the highest rate is obtained with p =16%. This feature can be understood in the following way: for a short sifted key X , an almost equally long string Z ( k ~ n ) is needed to reliably detect eavesdropping; when n grows, less bits of Z (in percentage) are necessary. In fact, in the large n limit, it is possible to choose k so that k / n vanishes as n goes to infinity and the secret key rate approaches the asymptotic bound, r =1− h 2 ( Q )− h 2 ( Q ). It is worth noting that, in the asymptotic limit, a biased choice of the bases gives a higher secure key rate with respect to the BB84 protocol [22] whenever p > . In fact, in the infinite limit, the fraction of secure over sifted bits is given by 1−2 h 2 ( Q ) in both cases (for simplicity we here assume ); however, a biased choice of the bases gives a number of sifted bits that is approximately >1/2 of the sent bits (also in the finite-size regime), whereas for the BB84 protocol the sifted bits are 1/2 of the sent bits. In particular, by using a large p , namely p ~1, in the infinite key limit we approach a double secret key rate with respect to BB84. In Fig. 2 the asymptotic bound of the secure key rate r , defined as the number of secure bits over number of sent bits, is twice the corresponding asymptotic bound of the BB84 protocol. With the obtained data, we also estimated the minimum number of received qubits M that are needed to obtain a key of given length . In Fig. 3 , we show this quantity as a function of the QBER (in this case, we assumed that Q = Q ). Solid lines represent the theoretical minimum M necessary to obtain a GS key for different lengths . With markers of different colours, we indicate the experimental received qubits for the different values of . Clearly, as the QBER grows, it is necessary to increase the number of exchanged qubits to obtain a given key length . On the other hand, when the channel is almost noiseless, a secret key of reasonable length can be extracted by using a relatively small number of qubits: for instance, more than 1,000 secure key bits can be obtained by exchanging <20,000 photons (see Fig. 3 ). 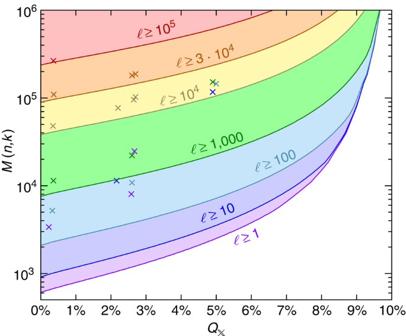Figure 3: Required bits for a secret key. Minimum number of received bitsM(n,k) needed to obtain aεsec−GS key of a given length(as labelled on each curve) versus the quantum BERQ. Different colours divide the regions with different secret key lengths. Crosses represent our experimental results, and the coloured regions and the solid lines that delimit them are derived from the numerically optimized bound, assumingQ=Q. Figure 3: Required bits for a secret key. Minimum number of received bits M ( n , k ) needed to obtain a ε sec −GS key of a given length (as labelled on each curve) versus the quantum BER Q . Different colours divide the regions with different secret key lengths. Crosses represent our experimental results, and the coloured regions and the solid lines that delimit them are derived from the numerically optimized bound, assuming Q = Q . Full size image In conclusion, we have experimentally demonstrated the feasibility of key distillation according to the finite-key analysis proposed in Tomamichel et al. [14] and compared it with a less stringent definition of security, called pragmatic, that protects the protocol against IS attacks. We compared the two analyses for different amounts of depolarizing noise added to the quantum channel. With pragmatic security, a significantly higher secret key rate with finite keys is demonstrated, even in conditions near the theoretical Q , Q bound of 11%. Its drawback is the insecurity against collective attacks, which however are not presently available. We stress that, when the channel is very noisy ( Q =8.3%), no key that is secure against the most general quantum attack could be extracted up to 2 × 10 5 sifted bits; however, by considering only IS attacks, in this case a secrect key rate up to 7.5% was obtained. When Q , Q >11%, it is not possible to obtain a secure key even in the asymptotic large n limit. This shows that, for highly noisy channels, the use of pragmatic secrecy is a viable solution to obtain some secret bits for an experimentally realistic number of exchanged photons. We believe that our work can have an important application for free-space quantum communication and for all QKD scenarios in which the number of exchanged qubits is limited by physical constraints, such as in the inter-satellite link scenario. Optical setup The optical setup of our prototype implementing the quantum communication is shown in Fig. 4 . The transmitter (Alice) uses four infrared (850 nm) attenuated diode lasers driven by a field programmable gate array (FPGA) to send the bits 0 and 1 encoded in the different polarization bases of the photons. By properly configuring the FPGA, it is possible to set the probabilities p and p . The receiver (Bob) uses a variable beam splitter (BS) with transmission T to send the received qubits to the measures in the two bases. The probability p is equal to the transmissivity T of the BS. On one BS output, a polarizing BS and two single-photon avalanche photodiodes measure the photons in the basis; on the other side, a half-wave plate is positioned before the polarizing BS to allow the measurement in the basis. The counts detected by the four single-photon avalanche photodiode are stored on a second FPGA. A cable between the two FPGA is also used along for synchronization. 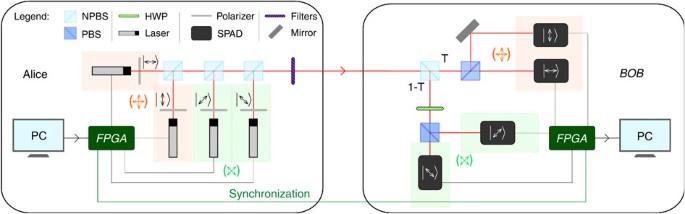Figure 4: Schematic representation of the experimental setup. The qubits are generated by attenuating four differently polarized lasers. At each qubit transmission the FPGA board controls which laser in turned on. At the receiver side, by a BS with transitivityT, Bob performs the measurement in the(with probabilityT) orbasis (with probability 1−T). Filters, neutral density filters; HWP, half-wave plate; NPBS, non-polarizing beam splitters; PBS, polarizing beam splitter; SPAD, single-photon avalanche photodiode. Figure 4: Schematic representation of the experimental setup. The qubits are generated by attenuating four differently polarized lasers. At each qubit transmission the FPGA board controls which laser in turned on. At the receiver side, by a BS with transitivity T , Bob performs the measurement in the (with probability T ) or basis (with probability 1− T ). Filters, neutral density filters; HWP, half-wave plate; NPBS, non-polarizing beam splitters; PBS, polarizing beam splitter; SPAD, single-photon avalanche photodiode. Full size image Concerning the transmitted qubits, we used the same data structure of a recent free-space QKD implementation [25] based on the B92 protocol [29] . A raw key is composed into N packets of 2,880 bits each, which are in turn divided into 12 frames for the ease of synchronization. In fact, each frame consists of 11 header slots and 240 payload slots, each with a duration of 800 ns. The header exhibits the pattern ‘100000xxxx1’, where ‘xxxx’ is the four-bit frame number, encoded one bit per slot in a pulse-duration modulation of the synchronization beam (a 400- or 200-ns pulse encode the bit 1 or 0, respectively). As regards the payload slots, the first 200 ns are used to send the synchronization signal; then, Alice waits for 200 ns and sends two bits separated by 200 ns. It is worth noting that the experimental setup of this protocol is very similar to the original BB84: the main difference lies in the interpretation of received bits in the two different bases. Classical post-processing After the parameter estimation phase, information reconciliation, error verification and privacy amplification are performed. Information reconciliation aims at correcting the discrepancies between X and X′ that the channel may have introduced, thus allowing Bob to compute an estimate of X . As a practical solution, we have chosen the Winnow scheme [30] that, by leveraging Hamming codes of different lengths over multiple iterations, allows an adaptive and lowly interactive error correction and represents a good trade-off between the high interactivity required by Cascade and the low flexibility of low density parity check (LDPC) code with limited key length. We fix an upper bound P fail to the probability of a reconciliation failure and, under this constraint, we optimize the parameters of the Winnow scheme to minimize the expected (average) classical information leakage [ L EC ]. First, given the average QBER on the basis Q , a threshold > Q is fixed so that the empirical QBER in the sifted key is higher than , with probability < P fail /2. Then, the block sizes are chosen so that the output BER is lower than P fail /(2 n ) whenever and [ L EC ] is minimized, as detailed in Canale et al. [25] Subsequently, an error verification mechanism such as the one proposed in Tomamichel et al. [14] ensures that the protocol is ε cor −correct, that is, that < ε cor , by comparing hashes of ([log 2 ( P fail / ε cor )]) bits. Namely, Alice chooses the hash function g randomly and uniformly from a class of universal 2 hash functions [31] (the class of Toeplitz matrices in our experimental setup) and computes her hash value g A = g ( X ). She then sends g A and a compact representation of g to Bob, who computes . The protocol aborts if the two hashes are different, that is, if g A ≠ g B . Finally, during the so-called privacy amplification, X and are compressed by means of a function that is, again, randomly and uniformly chosen from a class of universal 2 hash functions, to get the final secret keys S and . The length of the final key and the corresponding amount of compression depend on the required level of secrecy, the overall classical information leakage L EC +[log 2 ( P fail / ε cor )], the assumed attacker’s model and the estimate of the information leaked to the eavesdropper during the transmission over the quantum channel. Proof of pragmatic secrecy Proof of Theorem 1: let t be the number of qubits observed and measured by Eve on the basis among the n sifted bits. Then the Rényi entropy of order 2 for the sifted key, given all the information available to the eavesdropper, is lower-bounded by: being . Let us define the following pairs of complementary events, namely: let and be the aborting and non-aborting events, whereas R ={ R ( X | V )≥ n EC − a } and ={ R ( X | V )< n EC − a } define the events of acceptable and non-acceptable eavesdropping rate, respectively. Then, The multiplication of H ( S | V ) by the probability of not aborting yields Finally, by applying corollary 4 in Bennett et al. [32] to a possibly aborting protocol that outputs a bit key (that is, H ( U S )= ), we have, for every a , , From equation (12), we can upper bound the probability on the right-hand side of equation (16) as: because the two events in the right-hand side brackets of equation (17) refer to disjoint qubit sets, namely those encoded in the and basis, respectively, and are therefore independent. Furthermore, according to the selective individual attack model with attack rate q , t is a binomial random variable with parameters ( n , q ). Similarly, the number of measured errors on the basis, is a binomial random variable with parameters ( k , Q ) and Q = q /2. Therefore, we can rewrite equation (18) as: with F n , q (·) denoting the cumulative distribution function of a binomial random variable with parameters ( n , q ), and similarly for F k , q /2 (·). The last step is then assured by equation 6.6.4 in Abramowitz and Stegun [27] . Eventually, condition (5), together with definition (6) and given that , ensures that for any q ε[0,1] we get: Relationship between equations (1) and (3): the Pinsker inequality (see section 11.6 in Cover and Thomas [33] and Wilde [34] ) ensures that where u S is the uniform distribution on S and ( p || q ) is the relative entropy between the p and q distributions. By minimizing each term with respect to q V , we get: where equation (24) is because of ( p S V u S q V )= ( p S V u S q V )+ ( p V q V )≤ ( p S V u S p V ). It is then straightforward to see that: Relationship between equations (3) and (4): the uniformity condition trivially derives from the fact that H ( S | V )≤ H ( S ). Also, from basic information theory, we know that: because S has maximal entropy (that is, ) if and only if it is uniformly distributed. Now, because condition (3) is verified for any IS attack strategy, and therefore for any outcome V of the eavesdropper measurement on the quantum system E , the security condition directly follows. How to cite this article: Bacco, D. et al. Experimental quantum key distribution with finite-key security analysis for noisy channels. Nat. Commun. 4:2363 doi: 10.1038/ncomms3363 (2013).